Actomyosin-dependent formation of the mechanosensitive talin–vinculin complex reinforces actin anchoring The force generated by the actomyosin cytoskeleton controls focal adhesion dynamics during cell migration. This process is thought to involve the mechanical unfolding of talin to expose cryptic vinculin-binding sites. However, the ability of the actomyosin cytoskeleton to directly control the formation of a talin–vinculin complex and the resulting activity of the complex are not known. Here we develop a microscopy assay with pure proteins in which the self-assembly of actomyosin cables controls the association of vinculin to a talin-micropatterned surface in a reversible manner. Quantifications indicate that talin refolding is limited by vinculin dissociation and modulated by the actomyosin network stability. Finally, we show that the activation of vinculin by stretched talin induces a positive feedback that reinforces the actin–talin–vinculin association. This in vitro reconstitution reveals the mechanism by which a key molecular switch senses and controls the connection between adhesion complexes and the actomyosin cytoskeleton. During cell migration, focal adhesions (FAs) anchor the actomyosin cytoskeleton, organized in contractile stress fibres (SFs) in many cell types, to pull the cell body. FAs are clusters of transmembrane receptors of the integrin family that mechanically couple the actomyosin cytoskeleton to the extracellular matrix (ECM) via a variety of actin-binding proteins (ABPs) [1] . In response to the force generated by SFs, FAs undergo a compositional and morphological maturation during which regulatory proteins are recruited to reinforce the connection with the actomyosin cytoskeleton and the adhesion to the ECM [2] , [3] , [4] , [5] . The ABPs, vinculin and talin, play a central role during this process. In response to the force generated by the actomyosin cytoskeleton, vinculin accumulates in FAs where it transmits force [6] , [7] , [8] . Several FA proteins, including talin and the actin filament crosslinking protein α-actinin, interact with vinculin in vitro [9] , [10] , [11] . However, the localization of FA proteins along the vertical axis showed that vinculin colocalizes with talin, but not with α-actinin. α-actinin appears in an upper layer where it colocalizes with SFs [12] . In addition, the globular head domain of vinculin (Vh), which contains the talin-binding domain, is recruited to FAs [13] , while vinculin is not targeted to the membrane in cells lacking talin [14] . Although the mechanism by which vinculin is recruited to FAs is not fully understood, these observations support the view that talin plays a central role in this process. The actin-binding domain located in the vinculin tail (Vt) is masked by an intramolecular interaction with Vh [15] . The binding of talin to Vh induces a helical bundle conversion of this domain, leading to the release of Vt [16] . The simultaneous binding of talin to Vh and actin filaments to Vt facilitates the disruption of the autoinhibitory contacts [17] , [18] . Talin is one of the earliest ABPs to couple the actomyosin cytoskeleton to the ECM [19] . Talin contains three actin-binding domains (ABDs) located in the N-terminal FERM (four-point-one, ezrin, radixin, moesin) domain, the central part of the rod and the C-terminal part, respectively [20] ( Supplementary Fig. 1a ). The FERM domain also binds and contributes to activate integrins [21] . The rod domain contains 11 vinculin-binding sites (VBSs) [22] . Several of these VBSs are buried inside helix bundles [23] , [24] . Molecular dynamics simulations first predicted that the mechanical unfolding of a domain containing the first three helix bundles of the talin rod leads to the sequential exposure of VBSs [25] . The use of magnetic tweezers and atomic force microscopy showed that the stretching of a small fragment of the talin rod domain exposes cryptic VBSs, allowing the binding of several Vh molecules per talin [26] . Although the use of physical techniques revealed the mechanosensitive interaction between small fragments of talin and vinculin that do not interact with actin [26] , several issues remain open. Whether the direct binding of a contractile actomyosin network to talin is sufficient to stretch the protein and induce the association of vinculin has not been demonstrated. The reversibility of the force-dependent binding of vinculin to talin has never been tested. The parameters that govern the lifetime of the talin–vinculin complex have not been identified. Finally, whether the actomyosin-dependent activation of vinculin by talin, which releases the Vt domain, affects the dynamics of the actomyosin cytoskeleton is not known. To address these issues, we have developed a new microscopy assay with pure proteins in which the self-assembly of an actomyosin network, or SF-like cables, controls the association of vinculin to a talin-micropatterned surface in a reversible manner. This in vitro reconstitution of the actomyosin-dependent talin–vinculin complex reveals a mechanosensitive reinforcement of the association with the actin cytoskeleton. Actomyosin-dependent binding of vinculin to talin To determine whether the actomyosin cytoskeleton stretches talin to induce vinculin binding, we developed an in vitro assay with pure proteins ( Supplementary Fig. 1 ). In this microscopy assay, an actomyosin network generates force on talin-containing disc-shaped islands micropatterned on a glass coverslip ( Fig. 1 ). 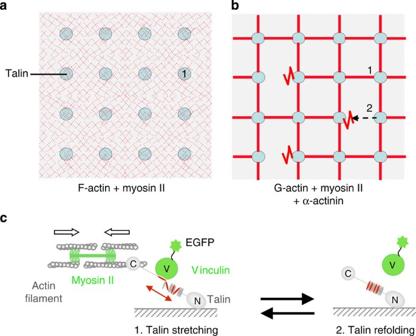Figure 1: Experimental strategies used in this study. (a) In this assay, a preformed actomyosin network (red), made of short actin filaments (F-actin) and myosin II filaments, generates force on talin-containing disc-shaped islands micropatterned on a glass coverslip. The force generated by this actomyosin network is sufficient to stretch talin and induce vinculin binding (see 1 in panelc). This experimental setup favours an instantaneous, homogeneous and synchronous mechanosensitive response. (b) Monomeric actin (G-actin), myosin II and α-actinin self-assemble into dynamic actomyosin cables (red) that control the association of vinculin to talin in a reversible manner. In these conditions, actomyosin cables stretch talin, allowing vinculin binding (see 1 in the panelc). The detachment of the cables allows vinculin dissociation and talin refolding (see 2 in the panelc). (c) Details of the reactions mentioned in (a) and (b). The mechanosensitive domain of talin corresponds to a group of helix bundles in the talin rod (amino acids 482–889) described in refs25,26. In talin, the vinculin-binding sites (VBSs) are in red and the other helices are in grey. Figure 1: Experimental strategies used in this study. ( a ) In this assay, a preformed actomyosin network (red), made of short actin filaments (F-actin) and myosin II filaments, generates force on talin-containing disc-shaped islands micropatterned on a glass coverslip. The force generated by this actomyosin network is sufficient to stretch talin and induce vinculin binding (see 1 in panel c ). This experimental setup favours an instantaneous, homogeneous and synchronous mechanosensitive response. ( b ) Monomeric actin (G-actin), myosin II and α-actinin self-assemble into dynamic actomyosin cables (red) that control the association of vinculin to talin in a reversible manner. In these conditions, actomyosin cables stretch talin, allowing vinculin binding (see 1 in the panel c ). The detachment of the cables allows vinculin dissociation and talin refolding (see 2 in the panel c ). ( c ) Details of the reactions mentioned in ( a ) and ( b ). The mechanosensitive domain of talin corresponds to a group of helix bundles in the talin rod (amino acids 482–889) described in refs 25 , 26 . In talin, the vinculin-binding sites (VBSs) are in red and the other helices are in grey. Full size image To determine the orientation of talin on the surface, we took advantage of the presence of calpain-2 cleavage sites in the protein [27] . In the assay, the cleavage of a C-terminally tagged talin-enhanced green fluorescent protein (EGFP) between amino acids Q433 and Q434 by a low concentration of calpain-2 ( Supplementary Fig. 2a,b ) provoked both the loss of the EGFP fluorescence and the dissociation of the actomyosin cytoskeleton from the discs ( Supplementary Fig. 2c,d ). In addition, actin was not recruited to the discs when the micropatterned surface was preincubated with a N-terminally deleted form of talin (482–2,541) ( Supplementary Fig. 2e ). Altogether, these results indicate that the N-terminal part of talin is bound to the surface, while its C-terminal ABD and/or its central ABD interact with actin filaments ( Supplementary Fig. 2f ). A similar orientation of talin was observed in FAs [12] . To follow the actomyosin-dependent talin–vinculin interaction in real time by total internal reflection fluorescence (TIRF) microscopy, we used the Vh domain fused with EGFP. In contrast with full-length vinculin, Vh interacts constitutively with talin VBSs. Since most of the VBSs are buried in the talin rod domain, Vh behaves as a conformation sensor that binds to newly exposed VBSs after talin stretching. We first used a contractile isotropic network made of prepolymerized short actin filaments and myosin II filaments to generate force on talin ( Fig. 1a,c ). This experimental setup favours an instantaneous, homogeneous and synchronous mechanosensitive response. In these conditions, we showed that the amount of Vh that accumulated in the discs was much higher in the presence of both actin and myosin than in the control experiment where actin or myosin was omitted ( Fig. 2a–g , Supplementary Movie 1 ). At saturating concentration of Vh, the steady-state fluorescence corresponding to talin-bound Vh was three times higher in the presence of both actin and myosin than in the control, demonstrating a force-dependent exposure of cryptic VBSs ( Fig. 2h ). The association rate of Vh to talin did not increase linearly with the concentration of Vh but reached a plateau, indicating that the force-dependent stretching of talin is a rate-limiting reaction ( Fig. 2i ). The exponential myosin dose dependence further suggests the existence of a threshold force to stretch talin ( Fig. 2j ). 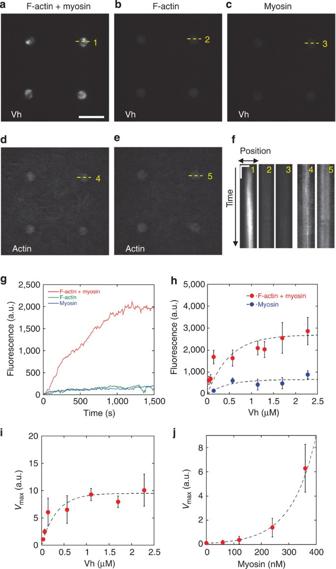Figure 2:In vitroreconstitution of the actomyosin-dependent binding of vinculin to talin. (a–f) Recruitment of Vh to talin-coated discs in the presence of an actomyosin network. Conditions: 22 nM of EGFP-Vh, 0.12 μM Myosin II, 2.4 μM of short actin filaments capped at their barbed end (2% Alexa594-labelled). The binding of EGFP-Vh and actin to talin-coated discs is shown at steady state in the presence of both actin and myosin (a,d), actin alone (b,e) and myosin alone (c). The pictures show EGFP-Vh (a–c) and actin (d,e). Scale bar, 15 μm.Supplementary Movie 1. (f) Kymographs of the cross-sections drawn in (a–e). Scale bar, 6 μm (horizontal), 300 s (vertical). (g) Kinetics of EGFP-Vh recruitment to talin-coated discs in the conditions described in the previous panels (a–f). (h) Steady-state fluorescence of talin-bound EGFP-Vh as a function of EGFP-Vh concentration in the presence of both actin and myosin or myosin alone as described in (a–f). Data are mean±s.d.,n≥8. Note that the experiment presented in (g) has been acquired with different camera settings and the fluorescence values cannot be compared with (h). (i) Maximum rate (Vmax) of EGFP-Vh binding to talin-coated discs as a function of EGFP-Vh concentration in the presence of actin and myosin as described in (a–f). Data are mean±s.d.,n≥8. (j) Maximum rate (Vmax) of EGFP-Vh binding to talin-coated discs, in the conditions described in (a–f), as a function of myosin concentration. Data are mean±s.d.,n≥8. (h–j), data collected in two independent experiments. Figure 2: In vitro reconstitution of the actomyosin-dependent binding of vinculin to talin. ( a – f ) Recruitment of Vh to talin-coated discs in the presence of an actomyosin network. Conditions: 22 nM of EGFP-Vh, 0.12 μM Myosin II, 2.4 μM of short actin filaments capped at their barbed end (2% Alexa594-labelled). The binding of EGFP-Vh and actin to talin-coated discs is shown at steady state in the presence of both actin and myosin ( a , d ), actin alone ( b , e ) and myosin alone ( c ). The pictures show EGFP-Vh ( a – c ) and actin ( d , e ). Scale bar, 15 μm. Supplementary Movie 1 . ( f ) Kymographs of the cross-sections drawn in ( a – e ). Scale bar, 6 μm (horizontal), 300 s (vertical). ( g ) Kinetics of EGFP-Vh recruitment to talin-coated discs in the conditions described in the previous panels ( a – f ). ( h ) Steady-state fluorescence of talin-bound EGFP-Vh as a function of EGFP-Vh concentration in the presence of both actin and myosin or myosin alone as described in ( a – f ). Data are mean±s.d., n ≥8. Note that the experiment presented in ( g ) has been acquired with different camera settings and the fluorescence values cannot be compared with ( h ). ( i ) Maximum rate ( V max ) of EGFP-Vh binding to talin-coated discs as a function of EGFP-Vh concentration in the presence of actin and myosin as described in ( a – f ). Data are mean±s.d., n ≥8. ( j ) Maximum rate ( V max ) of EGFP-Vh binding to talin-coated discs, in the conditions described in ( a – f ), as a function of myosin concentration. Data are mean±s.d., n ≥8. ( h – j ), data collected in two independent experiments. Full size image Tuning the stability of actomyosin cables by α-actinin To study the reversibility of the vinculin–talin complex, we modified the assay described previously in such a manner that this mechanosensitive interaction is controlled by a dynamic mechanical stimulus. We reconstituted the formation of dynamic SF-like cables in the presence of actin, myosin II and α-actinin ( Figs 1b and 3a and Supplementary Movie 2 ). To avoid the instant gelation of the actin network by α-actinin and favour the slow self-assembly of compacted cables, the components of the assay were mixed with monomeric actin (G-actin) in polymerizing conditions. The formation of compacted cables resulted from the contraction of the actomyosin network between two adjacent talin-coated discs ( Fig. 3b and Supplementary Movie 2 ). This first phase was followed by cycles of formation, detachment and retraction, reflecting cycles of isometric tension increase and release ( Supplementary Movie 2 ). To determine the effect of α-actinin on the tension applied by the cables on the talin-coated discs, we measured the retraction speed of detaching cables as a function of mCherry-α-actinin fluorescence along the cables. We found that the retraction speed was not affected by the density of mCherry-α-actinin, indicating that, in this range of concentrations, the crosslinking of actin filaments did not affect the tension applied on the talin-coated discs ( Fig. 3c–e , Supplementary Movie 3 ). However, we observed that increasing concentrations of α-actinin reduced the frequency of detachment ( Fig. 3f , Supplementary Movie 3 ). This last observation may reflect the ability of α-actinin to crosslink actin filaments of the tip of the cables with the rest of the actin network associated to the discs. Altogether, our observations indicate that α-actinin favours the establishment of a persistent isometric tension. 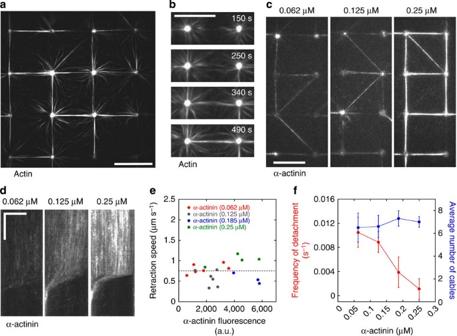Figure 3: α-actinin controls the stability of the actomyosin cables. (a) Self-assembly of actomyosin cables associated with talin-coated discs. Conditions: 2.4 μM G-actin (2% Alexa594-labelled), 0.12 μM Myosin II and 62 nM of α-actinin. Scale bar, 35 μm.Supplementary Movie 2. (b) Time lapse showing the formation of a cable between two talin-coated discs extracted from (a). Scale bar, 35 μm. (c) Self-assembly of actomyosin cables associated with talin-coated discs. Conditions: 2.4 μM G-actin, 0.12 μM Myosin II and the indicated concentrations of mCherry-α-actinin. Scale bar, 35 μm.Supplementary Movie 3. (d) Kymographs showing the retraction of mCherry-α-actinin-containing cables, at the indicated concentrations of mCherry-α-actinin. Scale bar, 10 μm (horizontal), 100 s (vertical). (e) Quantification of the retraction speed as a function of the fluorescence intensity of mCherry-α-actinin along the detaching cables, at the indicated concentrations of mCherry-α-actinin. (f) Quantification of the number of cables (in pictures showing 8 discs) and the frequency of detachment of the cables during time intervals of 400 s (in movies showing 8 discs) as a function of the concentration of mCherry-α-actinin. Data are mean±s.d. Number of cablesn≥20, frequency of detachmentn=6. Data collected in two independent experiments. The conditions for (d–f) are described in (c). Figure 3: α-actinin controls the stability of the actomyosin cables. ( a ) Self-assembly of actomyosin cables associated with talin-coated discs. Conditions: 2.4 μM G-actin (2% Alexa594-labelled), 0.12 μM Myosin II and 62 nM of α-actinin. Scale bar, 35 μm. Supplementary Movie 2 . ( b ) Time lapse showing the formation of a cable between two talin-coated discs extracted from ( a ). Scale bar, 35 μm. ( c ) Self-assembly of actomyosin cables associated with talin-coated discs. Conditions: 2.4 μM G-actin, 0.12 μM Myosin II and the indicated concentrations of mCherry-α-actinin. Scale bar, 35 μm. Supplementary Movie 3 . ( d ) Kymographs showing the retraction of mCherry-α-actinin-containing cables, at the indicated concentrations of mCherry-α-actinin. Scale bar, 10 μm (horizontal), 100 s (vertical). ( e ) Quantification of the retraction speed as a function of the fluorescence intensity of mCherry-α-actinin along the detaching cables, at the indicated concentrations of mCherry-α-actinin. ( f ) Quantification of the number of cables (in pictures showing 8 discs) and the frequency of detachment of the cables during time intervals of 400 s (in movies showing 8 discs) as a function of the concentration of mCherry-α-actinin. Data are mean±s.d. Number of cables n ≥20, frequency of detachment n =6. Data collected in two independent experiments. The conditions for ( d – f ) are described in ( c ). Full size image Talin refolding is limited by vinculin dissociation Although contractile actomyosin structures have been reconstituted recently [28] , [29] , the tunable dynamics of our assay offers the unique opportunity to observe the spatiotemporal coupling between the dynamics of actomyosin cables and the formation of the talin–vinculin complex. We showed that the association of cables with talin-coated discs was followed by the recruitment of Vh, while their frequent detachment was followed by the dissociation of Vh, reflecting the stretching and refolding of talin, respectively ( Fig. 4a–c , Supplementary Movie 4 ). To determine the hierarchy between talin refolding and vinculin dissociation, we compared the kinetics of Vh dissociation induced by the detachment of a cable ( k − =0.0035, s −1 , Fig. 4d , Supplementary Movie 4 ), and the kinetics of Vh dissociation from talin at steady state, measured by fluorescence recovery after photobleaching (FRAP), when an isotropic actomyosin network applies a constant force ( k − =0.0033, s −1 , Fig. 4d , Supplementary Fig. 3 , Supplementary Movie 5 ). The fact that the dissociation rate constant ( k − ) of Vh was not significantly affected by the irreversible refolding of talin indicates that talin refolding is kinetically limited by the dissociation of Vh. 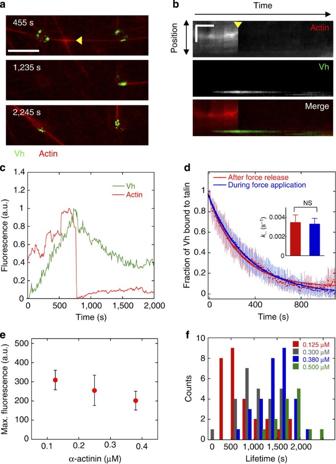Figure 4: Parameters that control the lifetime of the talin–vinculin complex. (a) Time lapse showing the colocalization of actomyosin cables and EGFP-Vh associated with talin-coated discs. Conditions: 22 nM of EGFP-Vh, 0.12 μM Myosin II, 2.4 μM of G-actin (2% Alexa594-labelled) and 0.12 μM α-actinin. Scale bar, 15 μm.Supplementary Movie 4. (b) Kymographs showing the detachment of the cable marked with an arrowhead in (a), followed by the dissociation of EGFP-Vh. Scale bar, 10 μm (vertical), 300 s (horizontal). (c) Quantification of the kymographs presented in (b). (d) Comparison between the kinetics of dissociation of EGFP-Vh from talin measured by FRAP when a constant force is applied (Supplementary Fig. 3c,d,Supplementary Movie 5) and after the detachment of a cable (conditions described inFig. 4a). Data were normalized between 1 and 0 to be compared. The inset shows a quantification of the dissociation rates. Data are mean±s.d. and theP-value was calculated (P=0.52) using at-test. Dissociation after force release,n=12; dissociation during force application,n=28. Data collected in three independent experiments. (e) Maximum intensity of EGFP-Vh fluorescence reached in the discs as a function of α-actinin concentration. Data are mean±s.d.,n≥32. Data collected in three independent experiments. (f) Distribution of the lifetime (time during which the intensity is 60% of the maximum) of EGFP-Vh spots associated with actomyosin cables as a function of α-actinin concentration. For (e) and (f), the conditions were described in (a). NS, not significant. Figure 4: Parameters that control the lifetime of the talin–vinculin complex. ( a ) Time lapse showing the colocalization of actomyosin cables and EGFP-Vh associated with talin-coated discs. Conditions: 22 nM of EGFP-Vh, 0.12 μM Myosin II, 2.4 μM of G-actin (2% Alexa594-labelled) and 0.12 μM α-actinin. Scale bar, 15 μm. Supplementary Movie 4 . ( b ) Kymographs showing the detachment of the cable marked with an arrowhead in ( a ), followed by the dissociation of EGFP-Vh. Scale bar, 10 μm (vertical), 300 s (horizontal). ( c ) Quantification of the kymographs presented in ( b ). ( d ) Comparison between the kinetics of dissociation of EGFP-Vh from talin measured by FRAP when a constant force is applied ( Supplementary Fig. 3c,d , Supplementary Movie 5 ) and after the detachment of a cable (conditions described in Fig. 4a ). Data were normalized between 1 and 0 to be compared. The inset shows a quantification of the dissociation rates. Data are mean±s.d. and the P -value was calculated ( P =0.52) using a t -test. Dissociation after force release, n =12; dissociation during force application, n =28. Data collected in three independent experiments. ( e ) Maximum intensity of EGFP-Vh fluorescence reached in the discs as a function of α-actinin concentration. Data are mean±s.d., n ≥32. Data collected in three independent experiments. ( f ) Distribution of the lifetime (time during which the intensity is 60% of the maximum) of EGFP-Vh spots associated with actomyosin cables as a function of α-actinin concentration. For ( e ) and ( f ), the conditions were described in ( a ). NS, not significant. Full size image Although a direct interaction between Vh and a single cryptic VBS in α-actinin has been reported [11] , we never detected the presence of EGFP-Vh along α-actinin-containing cables between two discs, and EGFP-Vh never followed a detaching cable ( Fig. 4a,b ). EGFP-Vh was only associated to the talin-coated surface. Therefore, in our assay, like in cells [12] , the role played by α-actinin in SFs is restricted to the crosslinking of actin filaments and its cryptic VBS is not exposed in this context. Mechanical stimulus duration sets talin–vinculin lifetime We determined how the α-actinin-dependent stability of the actomyosin cables affects the amplitude and the lifetime of the mechanosensitive response. Because the thin α-actinin-containing cables only cover a small fraction of the surface coated with talin, we restricted the quantification to the narrow region where the tip of the cable is attached to the disc. We found that increasing concentrations of α-actinin provoked a moderate reduction of Vh binding to talin ( Fig. 4e ). This effect may reflect the fact that, at high concentration of α-actinin, many crosslinked actin filaments are buried in the compacted cables and cannot interact with talin in the discs, hence reducing the number of talin-stretching events. Alternatively, this small effect could result from a competition between the two ABPs, α-actinin and talin, for actin filaments at the tip of the cables. The distribution of the lifetime of the talin–vinculin complex as a function of α-actinin concentration shows an increase from 250–500 s in the presence of 0.125 μM α-actinin to 1,750–2,000 s in the presence of 0.5 μM α-actinin ( Fig. 4f ). In agreement with our previous observations showing that α-actinin stabilizes the isometric tension applied by the cables ( Fig. 3e,f ), these observations show that α-actinin, by stabilizing the mechanical stimulus, indirectly extends the lifetime of the mechanosensitive talin–vinculin complex ( Fig. 4f ). A positive feedback stabilizes the actin–talin–vinculin link Finally, we determined whether the exposure of the actin-binding tail of activated vinculin (Vt) in talin-coated discs is sufficient to reinforce the connection with actin. We generated an autoinhibited EGFP-fused full-length vinculin (vinculin) that binds to actin filaments in a talin-dependent manner ( Supplementary Fig. 4c ). Like Vh, vinculin is recruited to talin-coated discs in an actomyosin-dependent manner ( Fig. 5a ). We compared the stability of the actomyosin cables anchored to talin-coated discs in the presence of Vh and vinculin. In this series of experiments, the discs were coated with a low concentration of talin to make the anchoring of the cable a limiting parameter. We also chose a high concentration of vinculin (2.2 μM) to favour the contribution of Vt. Finally, because α-actinin increases the stability of the cables, we performed these experiments in the presence of polymerizing actin and myosin only. In these conditions, loose cables assembled. In the presence of Vh, the system organized cables before it completely disorganized ( Fig. 5a,b,d , Supplementary Movie 6 ). In contrast, the binding of vinculin was followed by the continuous recruitment of actin filaments ( Fig. 5a,c,d , Supplementary Movie 6 ). Our observations demonstrate that the actomyosin-dependent activation of vinculin by talin induces a positive feedback that reinforces the actin–talin–vinculin association. 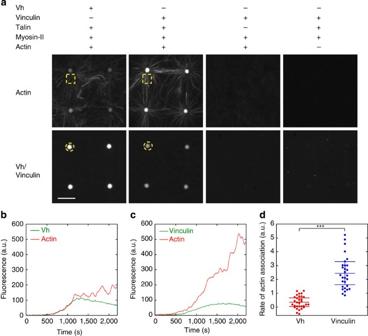Figure 5: A positive feedback stabilizes the actomyosin–talin–vinculin association. (a) Self-organization of actomyosin structures between talin-coated discs in the presence of EGFP-Vh and EGFP-vinculin as indicated. Conditions: 2.2 μM of EGFP-vinculin (or EGFP-Vh), 0.4 μM Myosin II, 1.2 μM of G-actin (2% Alexa594-labelled). In this series of experiments the discs are coated with a low concentration of talin (0.1 μM in the coating reaction) to make the anchoring of the cable a limiting parameter. Scale bar, 15 μm.Supplementary Movie 6. (b,c) Representative kinetics of EGFP-Vh/actin (b) and EGFP-vinculin/actin (c) binding to talin-coated discs. The regions of interest are indicated in (a). (d) Quantification of the rate at which actin is recruited to talin-coated discs after EGFP-Vh and EGFP-vinculin reached steady state (from 1,500 s to 2,200 s). Data are mean±s.d. For both EGFP-Vh and EGFP-vinculin,n=32 regions of interest collected in two independent experiments. TheP-value was calculated (P<0.0001) using at-test. Figure 5: A positive feedback stabilizes the actomyosin–talin–vinculin association. ( a ) Self-organization of actomyosin structures between talin-coated discs in the presence of EGFP-Vh and EGFP-vinculin as indicated. Conditions: 2.2 μM of EGFP-vinculin (or EGFP-Vh), 0.4 μM Myosin II, 1.2 μM of G-actin (2% Alexa594-labelled). In this series of experiments the discs are coated with a low concentration of talin (0.1 μM in the coating reaction) to make the anchoring of the cable a limiting parameter. Scale bar, 15 μm. Supplementary Movie 6 . ( b , c ) Representative kinetics of EGFP-Vh/actin ( b ) and EGFP-vinculin/actin ( c ) binding to talin-coated discs. The regions of interest are indicated in ( a ). ( d ) Quantification of the rate at which actin is recruited to talin-coated discs after EGFP-Vh and EGFP-vinculin reached steady state (from 1,500 s to 2,200 s). Data are mean±s.d. For both EGFP-Vh and EGFP-vinculin, n =32 regions of interest collected in two independent experiments. The P -value was calculated ( P <0.0001) using a t -test. Full size image In this study, we have developed a microscopy assay with pure components to demonstrate that the force generated by an actomyosin network on talin is sufficient to expose cryptic VBSs and induce vinculin binding. We have been able to reconstitute the spatiotemporal coupling between the formation and detachment of SF-like cables, the unfolding and refolding of talin and the resulting association and dissociation of vinculin. Kinetic analyses revealed that vinculin head dissociation limits talin refolding. By stabilizing actomyosin cables without affecting contractility, α-actinin increases the lifetime of the talin–vinculin complex. Finally, we showed that the actomyosin-dependent activation of vinculin by talin induces a positive feedback that reinforces the actin–talin–vinculin association ( Fig. 6 ). 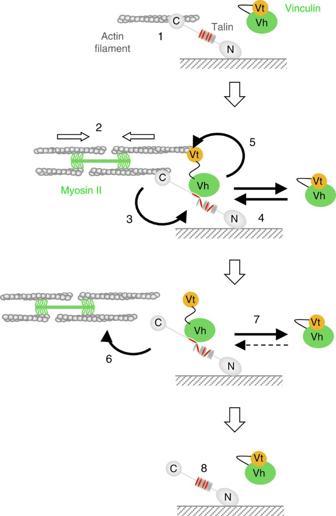Figure 6: Model for the actomyosin-dependent dynamics of the talin–vinulin complex. The mechanosensitive domain of talin is described at the end of the legend ofFig. 1. (1) Actin filament capture by talin. (2) Self-assembly of actomyosin cables. (3) Talin stretching, VBSs exposure. (4) Association and activation of vinculin. (5) Vinculin binding to actin and reinforcement of the anchoring. (6) Detachment of the cable. (7) Dissociation of vinculin. (8) Talin refolding, no reassociation of vinculin. Figure 6: Model for the actomyosin-dependent dynamics of the talin–vinulin complex. The mechanosensitive domain of talin is described at the end of the legend of Fig. 1 . (1) Actin filament capture by talin. (2) Self-assembly of actomyosin cables. (3) Talin stretching, VBSs exposure. (4) Association and activation of vinculin. (5) Vinculin binding to actin and reinforcement of the anchoring. (6) Detachment of the cable. (7) Dissociation of vinculin. (8) Talin refolding, no reassociation of vinculin. Full size image In cells, both the force applied on FAs and the myosin-dependent conformational dynamics of talin oscillate in periods ranging from a few seconds to minutes [30] , [31] . Efficient force transmission implies that the lifetime of the mechanosensitive complexes is controlled by reactions that limit protein refolding and stabilize force application. Our observations demonstrate that, in the case of the talin–vinculin complex, talin refolding is limited by the slow dissociation of vinculin head that follows the detachment of an actomyosin cable. In agreement with our observations, the overexpression of vinculin head (Vh) in living cells blocks the conformational dynamics of talin [30] . The stabilization of the stretched conformation of talin by Vh could also explain why the overexpression of Vh stabilizes FAs after myosin inhibition [32] . The slow dissociation rate of vinculin from talin is in agreement with previous in vitro studies [33] , but remains slower than vinculin dissociation from FAs [13] , [34] , suggesting that additional signals control the lifetime of this complex in vivo . In our model system, α-actinin does not affect the contractility of the SF-like cables but prevents their detachment, leading to a sustained formation of the talin–vinculin complex. Whether, in vivo , the primary role of α-actinin is to stabilize the connection between the actomyosin cytoskeleton and FAs to extend the lifetime of mechanosensitive complexes is not known. In favour of such an hypothesis, the centripetal elongation of FAs requires α-actinin to connect the growing adhesion plaque to the actin cytoskeleton [35] . Because cells lacking vinculin form FAs and SFs [36] , the importance of the actin-binding tail (Vt) of vinculin has long been elusive. However, recent studies showed that the actin-binding tail of vinculin is involved in the reorientation of FAs under force and controls the width of the lamellipodial actin network by slowing down the actin retrograde flow [32] , [37] . These observations may directly reflect our findings that the talin–vinculin complex senses the force through talin and responds by reinforcing its connection with actin through vinculin. In vivo , the use of a vinculin construct containing a FRET-based sensor between Vh and Vt demonstrated that vinculin transmits force in FAs [6] . Therefore, by providing a secondary path to transmit force to talin, activated vinculin could contribute to stretch talin and expose VBSs, leading to the recruitment of additional vinculin molecules. However, several observations in our assay rule out the existence of such an auto-amplification loop. First, vinculin fluorescence reached a plateau while actin continued to accumulate. In addition, vinculin and Vh reached a similar plateau at the same time ( Fig. 5b,c ). In conclusion, our study describes the molecular mechanism by which a key mechanosensitive switch senses and controls the connection between adhesion complexes and the actomyosin cytoskeleton. The assay presented here is a first step towards the in vitro reconstitution of more complex structures mimicking FAs and SFs. In particular, it would be interesting to determine how the diffusion of talin, bound to an integrin-containing lipid bilayer, affects the mechanosensitivity of the talin–vinculin complex. Our assay is also the ideal system to define the minimal set of SF proteins required to establish the sarcomeric-like structure of SFs in which α-actinin and myosin show a complementary periodic localization. Finally, this assay provides a new strategy to test the mechanosensitivity of a variety of ABPs associated with several cellular functions. Complementary DNA constructs pET-101-talin was constructed by PCR amplification of the human complementary DNA (cDNA) and direct subcloning of the resulting cDNA in the pET101/D-TOPO plasmid (Invitrogen). To generate the plasmid pET-101-talin-EGFP encoding for talin fused with EGFP at its C-terminus, the cDNA of EGFP was inserted into the Age I site of pET-101-talin. pGEX-6P2-mCherry-α-actinin-1, pGEX-6P2-α-actinin-1, pGEX-6P1-EGFP-vinculin-1-851 (Vh) and pGEX-6P1-EGFP-full-length-vinculin were constructed by PCR amplification of the human cDNAs and subcloning of the resulting cDNAs in the Eco RI and Not I sites of pGEX-6P2-mCherry, Eco RI and Not I sites of pGEX-6P2 (GE Healthcare), and Sal I and Not I sites of pGEX-6P1-EGFP (for vinculin 1–851 and full-length). pGEX-6P1-EGFP was a gift of Jan Faix (Hanover). pGEX-6P2-mCherry was constructed by PCR amplification of pmCherry (Clontech) and subcloning of the mCherry cDNA in pGEX-6P2 (GE Healthcare). All the constructs have been verified by sequencing. Protein purifications All the recombinant proteins were expressed using a similar protocol. First, the plasmid of interest was transformed in Escherichia coli (BL21 DE3, Invitrogen). Typically, transformed bacteria were grown in 4 l of LB medium containing 0.1 mg ml −1 of ampicillin at 37 °C until the absorbance at 600 nm reached 0.6–0.8. The culture was placed on ice until the temperature reached 16 °C. The expression of the recombinant protein of interest was induced by adding 0.5 mM isopropyl-β- D -thiogalactoside to the bacterial culture for 16 h at 16 °C. After centrifugation, the bacterial pellet was submitted to specific purification steps. Bacteria expressing talin or talin-EGFP were resuspended in lysis buffer (50 mM Tris pH 7.8, 500 mM NaCl, 5 mM Imidazole, 1 mM β-mercapto-ethanol) and sonicated. After high-speed centrifugation the clarified cell lysate was first submitted to Ni-NTA chromatography (HisTrap, GE Healthcare). The non-specifically bound proteins were removed by washing the column with 50 mM Tris pH 7.8, 500 mM NaCl, 30 mM Imidazole, 1 mM β-mercapto-ethanol, and the protein was eluted with a linear gradient of Imidazole (5–500 mM Imidazole). The buffer was then exchanged to 20 mM MES pH 6.3, 100 mM KCl, 1 mM β-mercapto-ethanol and the protein was applied to an ion exchange column (MonoQ 4,6/100 PE, GE Healthcare). The protein was eluted with a KCl gradient (100–500 mM). Finally, the protein was applied to a gel filtration column (Superdex 200 16/60, GE Healthcare) in 20 mM Tris pH 7.8, 150 mM KCl, 1 mM β-mercapto-ethanol. The purity of the protein was assessed by SDS–PAGE 4–15% (BioRad) ( Supplementary Fig. 1b ). The concentration of the protein was determined from the UV spectrum using a calculated extinction coefficient. The protein was finally supplemented with 200 mM sucrose as a cryoprotectant, frozen in liquid nitrogen and stored at −80 °C. Bacteria expressing full-length α-actinin, mCherry-α-actinin, EGFP-vinculin 1–851 (Vh) and EGFP-vinculin were resuspended in lysis buffer (50 mM Tris pH 7.8, 500 mM NaCl, 1% Triton X-100 and 1 mM dithiothreitol (DTT)) and sonicated. After high-speed centrifugation (30,000 g ), cell lysate was first incubated with glutathione sepharose (GE Healthcare). After 2 h of incubation at 4 °C, the resin was washed with 50 mM Tris pH 7.8, 500 mM NaCl and 1 mM DTT. The protein of interest bound to the resin was cleaved from the glutathione S -transferase (GST) tag by adding the GST-fused PreScission protease (GE Healthcare) in cleavage buffer (50 mM Tris pH 7.8, 150 mM NaCl, 1 mM EDTA, 1 mM DTT). The eluted protein was collected by low-speed centrifugation (5,000 g ). mCherry-α-actinin was further purified by gel filtration chromatography (Superdex 200, 16/60, GE Healthcare) in 50 mM Tris pH 7.8, 150 mM NaCl, 1 mM EDTA, 1 mM DTT. mCherry-α-actinin was finally applied to an ion exchange column (MonoQ, 4,6/100 PE, GE Healthcare) in 20 mM Tris pH 7.9, 150 mM NaCl, 1 mM CaCl 2 , 5 mM β-mercapto-ethanol and eluted with a NaCl gradient (50–1000, mM). Finally α-actinin and mCherry-α-actinin were dialysed in 20 mM Tris pH 8, 150 mM KCl, 1 mM CaCl 2 , 5 mM β-mercapto-ethanol. EGFP-vinculin was further purified by gel filtration chromatography (Superdex 200, 16/60, GE Healthcare) in 20 mM Tris pH 7.5. EGFP-Vh and EGFP-vinculin were dialysed in 20 mM Tris pH 7.8, 100 mM KCl. All the proteins were ultracentrifuged at 300,000 g in a TL100 (Beckman) to remove aggregates and test their solubility. The purity was assessed by SDS–PAGE 4–15% (BioRad) ( Supplementary Fig. 1b ). The concentration of the proteins was determined from the UV spectrum using extinction coefficients. Finally, the proteins were frozen in liquid nitrogen and stored at −80 °C. Talin 482–636 (VBS1) was expressed as a GST fusion protein in E. coli BL21, bound to glutathione sepharose (GE Healthcare), and finally eluted by PreScission protease (GE Healthcare) cleavage [17] . Actin was extracted from rabbit skeletal muscle acetone powder and submitted to cycles of polymerization and depolymerization [38] . Finally, actin was gel filtered through a Superdex G-200 column (GE Healthcare) in 5 mM Tris pH 7.8, 0.1 mM CaCl 2 , 0.2 mM ATP, 1 mM DTT. Purified monomeric Ca-G-actin (calcium-bound monomeric actin) was kept on ice. Actin was labelled on lysines with succinimidyl-ester Alexa594 (Invitrogen). Myosin II was extracted from rabbit skeletal muscle. Briefly, myosin is extracted from ground muscle in 0.5 M KCl, 0.1 M K 2 HPO 4 . After centrifugation, the actin-containing pellet is discarded, while the myosin-containing supernatant is further purified. Myosin was submitted to several cycles of precipitation by dilution in water or low-ionic-strength buffers, followed by centrifugation and resuspension in high-salt buffers [39] , [40] . Myosin was finally dialysed in 20 mM KH 2 PO 4 /K 2 HPO 4 pH 7.5, 0.5 M KCl, 1 mM EDTA, supplemented with 50% glycerol and stored at −20 °C. Several studies have reported protocols to extract and purify talin, vinculin and α-actinin from smooth muscle [41] , [42] , [43] , [44] , [45] . Recombinant vinculin, expressed in E. coli , has also been purified [46] . In order to purify recombinant proteins tagged with EGFP and mCherry, expressed in E. coli , we developed protocols that differ from the well-established ones mentioned above. Although Triton X-100 is not necessary to purify these proteins from tissues, as demonstrated for vinculin for example [45] , this detergent was added during the bacterial lysis step to help cell permeabilization and reduce non-specific binding to resins used for affinity chromatography. All our purification protocols include extensive washes and chromatography steps that efficiently eliminate traces of Triton X-100 from the proteins. We performed several experiments to test the effect of the fluorescent tags and the purification conditions on the activity of the recombinant proteins. The crosslinking activity of α-actinin and mCherry-α-actinin was measured by right angle light scattering at 350 nm in a fluorimeter (Xenius, Safas, Monaco). We found that mCherry does not affect the crosslinking activity of α-actinin ( Supplementary Fig. 4a ). We verified that the presence of Triton X-100 during the lysis step does not affect the final activity of α-actinin and mCherry-α-actinin ( Supplementary Fig. 4a ). We also verified that the presence of Triton X-100 during the lysis step does not affect the ability of EGFP-Vh to interact with talin-coated discs in the presence of actin and myosin ( Supplementary Fig. 4b ). Finally, we verified that EGFP-fused full-length vinculin is autoinhibited by a Vh–Vt intramolecular interaction and that the binding of the VBS1 domain of talin (talin 482–636) to Vh provokes the release of Vt. Talin VBSs interact with fully exposed Vh with high affinity ( K d =15–80 nM), while VBSs interact weakly, or not, with autoinhibited vinculin ( K d >25 μM) [15] , [17] . However, in conditions where VBSs induce vinculin binding to actin filaments, the affinity of VBSs for vinculin is increased because both VBSs and actin filaments stabilize the activated form of vinculin. FRET measurements showed that vinculin binds a VBS peptide or the talin rod domain, in the presence of actin, with K d values of 0.48 and 2.9 μM, respectively [18] . Similarly, we previously showed that, in a F-actin cosedimentation assay, VBS1 interacts with non-tagged vinculin, purified in the absence of Triton X-100, with a K d of 5 μM [17] . Therefore, our observation showing that VBS1 induces the cosedimentation of EGFP-vinculin with actin filaments with a K d of 1.5 μM demonstrates that EGFP-vinculin used in this work displays the expected features of autoinhibited vinculin ( Supplementary Fig. 4c ). Sample preparation for the in vitro assay This assay is based on the use of a micropatterned surface. This surface is a glass coverslip passivated with polyethylene glycol (PEG) or an equivalent compound that is locally removed by UV irradiation through a mask to draw specific patterns [28] , [47] . Here we use coverslips covered by discs of 6 μm in diameter, regularly spaced by 35 μm, provided by Cytoo (Grenoble, France). The flow chamber was made of a micropatterned coverslip 20 mm × 20 mm attached to a glass slide (Super Frost, Agar, Oxford Instruments) with two bands of 0.4 mm thick double-sided adhesive tape. The volume of a typical chamber was 100 μl (20 mm × 13 mm × 0.4 mm). The chamber was first incubated with talin (0.5 μM) in F-buffer (10 mM Tris pH 7.8, 25 mM KCl, 1 mM MgCl 2 , 0.2 mM CaCl 2 , 1 mM DTT, 1% BSA) for 5 min at room temperature. The excess of unbound talin was washed out with 200 μl of F-buffer. The surface of the discs was passivated by incubating the chamber with 100 μl of F-buffer containing BSA (10%) and casein (10 mg ml −1 ) for 5 min at room temperature and washed with 200 μl of F-buffer. Finally, 100 μl of the reaction was added to the chamber. A typical reaction was prepared by adding 0.12 μM myosin II, 2.4 μM Ca-G-actin, 1% BSA, 0.5 mg ml −1 casein and an ATP regenerating mix (2 mM ATP, 2 mM MgCl 2 , 10 mM creatine phosphate, 3.5 U ml −1 creatine kinase) in G-fluo buffer (10 mM Tris pH 7.8, 0.2 mM CaCl 2 , 0.4% methylcellulose, 5 mM DABCO and 20 mM DTT). Finally, 2 mM MgCl 2 and 0.2 mM EGTA were added to the reaction to transform Ca-G-actin into Mg-G-actin (magnesium-bound monomeric actin), and 25 mM KCl was added to the reaction to induce actin polymerization. Importantly, this low ionic strength allows myosin to form bipolar filaments. After the reaction was injected, the flow chamber was sealed with VALAP (a mixture of vaseline, lanolin and paraffin wax). Additional proteins such as α-actinin, mCherry-α-actinin, EGFP-Vh and EGFP-vinculin were also added. The short actin filaments used in several reactions were prepared by mixing prepolymerized actin with the barbed-end capping protein gelsolin at a 1:2,000 gelsolin/actin molar ratio. TIRF microscopy and data analysis The assay described in the previous section was observed by TIRF microscopy. TIRF images were acquired with an Olympus IX71 inverted microscope equipped with an oil 60 × objective (1.45 NA) (Olympus). EGFP-vinculin was excited with the 473 nm laser (Cobolt), and Alexa594-labelled actin and mCherry-α-actinin were excited with a 561 nm laser (Cobolt). The time-lapse videos were acquired with a Cascade II camera (Photometrics) controlled by Metamorph and subsequently analysed by the ImageJ software. Kymographs were generated in Image J by using the ‘Kymo Tool Box’ plugin. FRAP experiments FRAP experiments were performed to measure the rate constant of fluorescence recovery of EGFP-Vh bound to talin. The experiments were performed as soon as the kinetics of EGFP-Vh binding to talin-coated discs reached the plateau (steady-state) in the presence of myosin and short actin filaments capped at their barbed ends. FRAP experiments were first performed on a spinning disk confocal microscope setup (Nikon TIE) using a 60 × Plan APO objective (1.49 NA) and a FRAP module equipped with a 491 nm laser (iLas [2] , Roper Scientific SARL, Evry, France). Circular regions (10 μm in diameter) were drawn around the discs and bleached by 20 iterative pulses of 20 ms each using the 491 nm laser at 50% power. FRAP was monitored on a single plane for 1,500 s (1 frame per 10 s) using the 491 nm laser at 9.5% power. We bleached 70±5% of the fluorescence and observed a 72±4% recovery. The fluorescence of nonbleached discs did not change during the recovery of the bleached discs. The rate constant of recovery was slow ( k =0.0029±0.0005, s −1 , mean±s.d., n =6, data collected in two independent experiments, Supplementary Fig. 3a,b ). This rate was very similar to the rate at which Vh dissociates after a cable detaches ( k =0.0034±0.0007, s −1 , mean±s.d., n =12, data collected in three independent experiments, Fig. 4d ), derived from TIRF microscopy observations. To obtain the most accurate comparison of the two rate constants, presented in the Fig. 4d , we measured them with the same experimental setup. We performed FRAP experiments with the TIRF microscope that we used to observe the dissociation of Vh induced by the detachment of cables ( Fig. 4a–d ). Although our TIRF microscope was not equipped with a conventional FRAP system, the slow fluorescence recovery allowed us to bleach the initial fluorescence by a 1,000 ms continuous illumination of the surface with the evanescent wave generated by the 473 nm laser. Recovery was monitored for 1,500 s (1 frame per 10 s, 20 ms exposure time). We bleached 70±9% of the fluorescence and observed an 80±9% recovery. The rate constant of recovery measured on the TIRF microscope ( k =0.0033±0.0006, s −1 , mean±s.d., n =28, data collected in three independent experiments, Fig. 4d , Supplementary Fig. 3c,d , Supplementary Movie 5 ) was similar to the rate constant measured on the spinning disk microscope mentioned earlier ( k =0.0029±0.0005, s −1 , mean±s.d., n =6, data collected in two independent experiments, Supplementary Fig. 3a,b ). In preliminary attempts, we determined that the maximum rate of recovery was observed at 0.5 μM EGFP-Vh. On the basis of this observation, we chose to perform the FRAP experiments at 1 μM EGFP-Vh. In these conditions the fast reassociation is not a limiting parameter. The rate of fluorescence recovery is only limited by the dissociation rate of the bleached EGFP-Vh molecules from talin. Therefore we interpreted the rate constant of fluorescence recovery ( k ) as a dissociation rate constant ( k − ) and compared it with the dissociation rate constant of Vh from talin-coated discs after the detachment of actomyosin cables ( Fig. 4d ). Importantly, we observed that the final level of fluorescence recovery was affected by the laser power on the spinning disk confocal microscope and by the illumination time on the TIRF microscope used to bleach the initial fluorescence. None of the two setups allowed us to bleach 100% of the signal with a 100% recovery. For example, on the TIRF microscope, a mild bleaching of 55% of the initial fluorescence lead to a 95% recovery, while a strong bleaching of 80% of the initial fluorescence lead to a 70% recovery. However, the rate constants of recovery were not different. Therefore, the fraction of fluorescence that does not recover most likely corresponds to the photodamaged fraction of the talin-coated surface during the photobleaching. FRAP analysis was performed with ImageJ. The background was first subtracted. The average fluorescence of the discs was measured. The ratio postbleach/prebleach was calculated. The fluorescence recovery kinetics were analysed using Kaleidagraph, and a single exponential equation was used to fit the data: F ( t )=( F ma x − F min )(1− e − kt )+ F min , where F(t) is the normalized fluorescence intensity at time t , F max and F min are the maximum and minimum fluorescence after bleaching and k is the rate constant of fluorescence recovery. The kinetics of fluorescence recovery measured on the TIRF microscope were also normalized between 1 and 0 to be compared with the dissociation kinetics of EGFP-Vh from talin measured after the detachment of an actomyosin cable ( Fig. 4d ). How to cite this article: Ciobanasu, C. et al. Actomyosin-dependent formation of the mechanosensitive talin–vinculin complex reinforces actin anchoring. Nat. Commun. 5:3095 doi: 10.1038/ncomms4095 (2014).